Ferroelectric tunnel junctions with graphene electrodes Polarization-driven resistive switching in ferroelectric tunnel junctions (FTJs)—structures composed of two electrodes separated by an ultrathin ferroelectric barrier—offers new physics and materials functionalities, as well as exciting opportunities for the next generation of non-volatile memories and logic devices. Performance of FTJs is highly sensitive to the electrical boundary conditions, which can be controlled by electrode material and/or interface engineering. Here, we demonstrate the use of graphene as electrodes in FTJs that allows control of interface properties for significant enhancement of device performance. Ferroelectric polarization stability and resistive switching are strongly affected by a molecular layer at the graphene/BaTiO 3 interface. For the FTJ with the interfacial ammonia layer we find an enhanced tunnelling electroresistance (TER) effect of 6 × 10 5 %. The obtained results demonstrate a new approach based on using graphene electrodes for interface-facilitated polarization stability and enhancement of the TER effect, which can be exploited in the FTJ-based devices. One of the most promising aspects of ferroelectric research, which has recently drawn a lot of attention, is the effect of resistive switching associated with electrically or mechanically induced polarization reversal [1] , [2] , [3] , [4] , [5] , [6] . In addition to being highly relevant to technological applications in memory and logic devices, it concerns the fundamental issues of the critical behaviour and switching dynamics in ultrathin ferroelectric films, role of structural defects in the transport properties and scalability of these structures at the nanoscale. Earlier reports on the transport behaviour of relatively thick ferroelectric films (>50 nm) considered several possible mechanisms, such as Poole–Frenkel conduction [7] , Fowler–Nordheim tunnelling [8] , thermionic emission [9] and Schottky barrier variations [10] . Advances in fabrication of epitaxial ferroelectric films with the thickness of just several unit cells allowed realization of electron transport via the direct tunnelling mechanism. It has been theoretically predicted that reversal of the polarization in ferroelectric tunnel junctions (FTJs) utilizing such ultrathin films would change the potential barrier between the electrodes and, hence, alter the transmission probability resulting in the tunnelling electroresistance (TER) effect [5] , [11] , [12] . Experimental studies of TER showed that the difference between the high- and low-conductance states (ON and OFF states) associated with opposite polarization directions could reach several orders of magnitude [2] , [13] , [14] . It has been also found that the film–electrode interface properties play a critical role in the TER effect, resulting in tunable resistivity and affecting polarization retention [15] , [16] , [17] . Ionic displacement and orbital hybridization at the interfaces, non-stoichiometry and charge defects affect the boundary conditions, which determine the potential barrier profile. Most recently it has been demonstrated that significant enhancement of the electroresistance effect can be achieved by using a semiconducting material as one of the FTJ’s electrodes [3] . In this case, the TER enhancement is a result of switching between accumulation and depletion of the majority carriers at the semiconductor interface due to a ferroelectric field effect. Another approach makes use of the ferroelectrically induced metal–insulator transition in the interfacial oxide layer pushing the TER ratio even higher [18] . These observations show that the interface engineering is an efficient way to amplify the resistive switching effect in FTJs. One of the particularly attractive approaches to realize interface engineering is through the introduction of molecular layers (MLs) with certain characteristics at the electrode–ferroelectric interface. Considering a practically infinite number of available molecules with a wide range of variable parameters, such as size, shape, dipole moment and so on, this approach may provide abundant possibilities to tune the electrical properties of FTJs. However, practical realization of an FTJ with controllable interfacial ML is very challenging and has not been demonstrated yet. In ambient conditions, achieving a stable ML on the surface of a ferroelectric film is difficult due to the presence of dynamic surface adsorbates, such as water molecules, which means that the ML should be stabilized with a top electrode. However, deposition of an electrode material is typically performed under vacuum, which would result in ML desorption. In this study, we demonstrate that the interfacial ML engineering could be achieved by using graphene, a two-dimensional carbon allotrope [19] , as a top electrode of a FTJ. Graphene, which allows a wide-range modulation of its electronic properties via a field-effect approach, is currently being actively employed in advanced functional devices, such as ferroelectric field-effect transistors [20] , [21] , [22] . However, while the previous studies of graphene–ferroelectric structures were focused on the modulation of the in-plane conductivity, graphene has never been proposed as an electrode material in FTJs for measurements of perpendicular-to-the-plane transport. Graphene is impermeable for any gas or liquid, suggesting that it could be used to trap and stabilize any molecules on the ferroelectric surface [23] , [24] , [25] . The ease with which graphene can be transferred on any surface opens a possibility of using it in various devices with engineered interfaces, including FTJs. High-quality graphene sheets of practically any size could be conveniently synthesized on copper foils by the chemical vapour deposition (CVD) method and then transferred to the surface of a ferroelectric film by a wet chemistry procedure [26] , [27] . As we demonstrate in this paper, MLs could be easily introduced to the graphene/ferroelectric interface providing a simple and straightforward method to fabricate FTJs with enhanced performance characteristics. Interface engineering We realize this approach by using ferroelectric BaTiO 3 (BTO)-based tunnel junctions with graphene top and (La,Sr)MnO 3 bottom electrodes. Epitaxial single-crystalline BTO films with the thickness of 6 unit cells (u.c.) have been fabricated by pulsed layer deposition on epitaxial La 0.67 Sr 0.33 MnO 3 (LSMO) layers grown on atomically smooth (001) SrTiO 3 (STO) substrates [28] (see Methods for details). This type of substrate is known to produce compressively strained BTO films that possess only out-of-plane polarization [29] . Engineering of the graphene–ferroelectric interfaces has been realized by introducing an additional ML formed during the transfer of graphene to the ferroelectric surface in different solvents. Specifically, we have incorporated H 2 O or NH 3 layers at the graphene/BTO interfaces ( Fig. 1a ). Details of the processing method are described in Methods. Briefly, the 10 × 30-μm 2 graphene patches were fabricated by a combination of e-beam lithography and reactive ion etching on the SiO 2 /Si wafer, which was subsequently spin-coated by poly(methyl methacrylate) (PMMA) and placed on the surface of HF solution to etch away SiO 2 . Introduction of the ammonia or water layer at the graphene/BTO interface was achieved by washing the PMMA/graphene film in water (H 2 O sample) or with ammonium hydroxide solution (NH 3 sample) followed by its transfer to the BTO surface after which the PMMA layer was removed by acetone. From here on, we denote junctions with graphene patches transferred in ammonia and water as Gr/NH 3 /BTO and Gr/H 2 O/BTO, respectively. 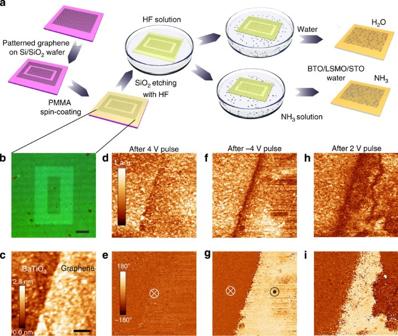Figure 1: Sample preparation and PFM testing of the switching behaviour of the Gr/NH3/BTO/LSMO junctions. (a) Schematics of the steps for sample preparation (see text for details). (b) An optical image of the 10 × 30-μm2graphene patch. (c) Topographic image of the edge of the graphene patch along with the segment of the bare BaTiO3surface. (d–i) PFM amplitude (d,f,h) and phase (e,g,i) images of the Gr/NH3/BTO/LSMO junction after application of 4 V (d,e), −4 V (f,g) and 2 V (h,i) pulses, showing changes of the domain structures under graphene. Scale bar, 10 μm (b) and 0.2 μm (g). Figure 1: Sample preparation and PFM testing of the switching behaviour of the Gr/NH 3 /BTO/LSMO junctions. ( a ) Schematics of the steps for sample preparation (see text for details). ( b ) An optical image of the 10 × 30-μm 2 graphene patch. ( c ) Topographic image of the edge of the graphene patch along with the segment of the bare BaTiO 3 surface. ( d – i ) PFM amplitude ( d , f , h ) and phase ( e , g , i ) images of the Gr/NH 3 /BTO/LSMO junction after application of 4 V ( d , e ), −4 V ( f , g ) and 2 V ( h , i ) pulses, showing changes of the domain structures under graphene. Scale bar, 10 μm ( b ) and 0.2 μm ( g ). Full size image Ferroelectric switching and retention First, we tested the reliability of electrical control of polarization in the FTJ with the graphene top electrode by performing piezoresponse force microscopy (PFM) imaging of the polarization states through the 10 × 30-μm 2 graphene patches ( Fig. 1b ) before and after voltage pulse application. Figure 1c shows the topographic image of the edge of the graphene patch (on the right) on the bare BTO surface (on the left). PFM testing of the FTJs shows that as-grown BTO films are in a single-domain state with polarization oriented downwards (towards the bottom interface). Polarization states resulting from application of the voltage pulses by the PFM tips in contact with the graphene patch are shown in Fig. 1d–i . It can be clearly seen that polarization can be switched either completely or in small fractions depending on the pulse amplitude (or duration), indicating an efficient polarization control with external voltage. Note that polarization state of the exposed BTO film remains unchanged. Polarization switching in the FTJs was also confirmed by PFM hysteresis loop measurements (see Supplementary Fig. 1 ; Supplementary Note 1 ). Similar switching behaviour has been observed in all types of samples including the reference ones where graphene was deposited directly on the BTO surface (Gr/BTO/LSMO junctions) without addition of the interfacial layer ( Supplementary Fig. 1 ). As for polarization retention, we found that introduction of the NH 3 layer results in a much more stable polarization (with retention time of at least several days for both polarization states), as compared with the FTJs with the H 2 O layer where only one stable polarization state (downwards) can be observed ( Supplementary Figs 2 and 3 ; see also Supplementary Note 2 ). Note that the instability of the upward polarization state has been also observed in the Gr/BTO/LSMO junctions ( Supplementary Fig. 4 ), which rules out the effect of the graphene electrode and emphasizes a decisive role of the interfacial layer in polarization retention. Testing of resistive switching Next, we characterized the resistive switching behaviour by measuring the current–voltage ( I – V ) characteristics of the FTJs as a function of their polarization state using the conductive-atomic force microscopy approach. Given its superior retention properties, we have focused on the Gr/NH 3 /BTO junctions. 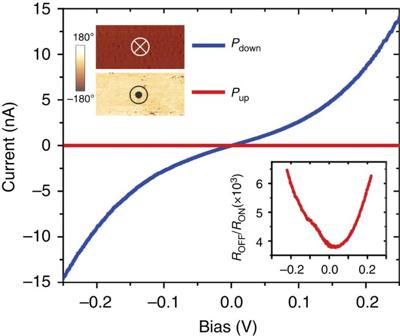Figure 2: Electroresistance effect in the Gr/NH3/BTO/LSMO junctions. TheI–Vcurves measured for the upward (red) and downward (blue) BaTiO3polarization states. The lower-right inset shows that theROFF/RONresistance ratio is about 3,800 for a zero-bias regime and increases up to 6,000 for ±0.2 V. The upper-left inset shows the PFM images of the upward and downward polarization states after theI–Vtesting, illustrating that polarization is not affected by theI–Vmeasurements. Figure 2 shows the I – V curves measured after complete switching of the BTO polarization either up or down by applying the ±4 V voltage pulses. It is seen that there is a giant resistance change upon polarization reversal: the OFF/ON ratio R OFF / R ON reaches a factor of >3,800 in the zero-bias limit and can be as large as 6,000 for the bias range of ±0.2 V. This effect is much stronger than that reported earlier for bare BTO films of the same thickness (6 u.c.) with the TER magnitude of about 7 (ref. 13 ). Note that the observed I – V curves of both polarization states can be fitted exceptionally well using the Brinkman’s model [30] (see Supplementary Fig. 5 ), yielding realistic barrier parameters. This finding suggests that the tunnelling mechanism provides a realistic description of the observed transport phenomena. (Further details can be found in Supplementary Note 3 .) The observed effect is highly reproducible and stable: the I – V curves measured at different locations on the surface of the graphene patch display similar behaviour and show no degradation within the period of polarization stability (that is, for at least several days). In addition, conductive-atomic force microscopy measurements performed on the junctions fabricated using several different BTO/LSMO substrates show little junction-to-junction variations ( Supplementary Note 4 ). To test the electrical endurance, the Gr/NH 3 /BTO/LSMO junctions have been subjected to repetitive switching. No significant degradation of the switchable polarization and electroresistance effect has been observed after ~4 × 10 3 switching cycles ( Supplementary Fig. 6 ). Figure 2: Electroresistance effect in the Gr/NH 3 /BTO/LSMO junctions. The I – V curves measured for the upward (red) and downward (blue) BaTiO 3 polarization states. The lower-right inset shows that the R OFF / R ON resistance ratio is about 3,800 for a zero-bias regime and increases up to 6,000 for ±0.2 V. The upper-left inset shows the PFM images of the upward and downward polarization states after the I – V testing, illustrating that polarization is not affected by the I – V measurements. Full size image The obtained results suggest that the electrode/ferroelectric interface properties play a crucial role in the polarization-induced resistive switching behaviour in FTJs. Introduction of the NH 3 layer at the graphene/BTO interface not only stabilizes the polarization of BTO but also significantly enhances the TER effect. The difference in polarization retention between the Gr/H 2 O/BTO and Gr/NH 3 /BTO junctions can be explained by considering the electronic structure of the water and ammonia molecules. According to the valence shell electron–pair repulsion (VSEPR) theory [31] , the water molecule has four, approximately tetrahedrally arranged, sp 3 -hybridized electron pairs, two of which are associated with bonding between O and H atoms and the other two are lone pairs on the oxygen ( Fig. 3a ). This arrangement gives rise to a dipole moment with the polar vector bisecting the H–O–H angle. Similarly, the ammonia molecule has a tetragonal arrangement of electron pairs with three pairs bonding three hydrogen atoms with nitrogen leaving it with one lone pair ( Fig. 3b ). The dipole moment vector of the ammonia molecule coincides with this lone pair. Below we describe, on the basis of the VSEPR theory, how polarization of the TiO 2 -terminated BTO layer affects the orientation of dipole moments of water and ammonia molecules at the graphene/BTO interface, which in turn affects the BTO polarization retention. 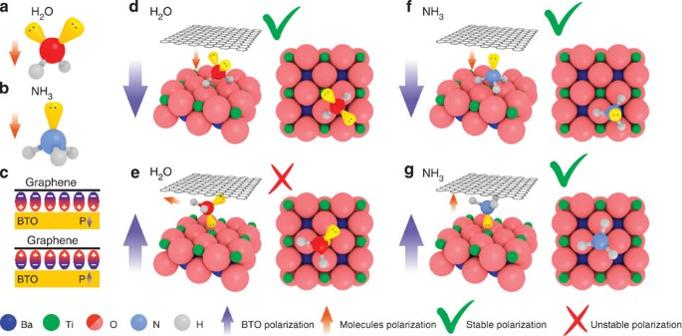Figure 3: Differences in the alignment of water and ammonia molecules at the graphene/BTO interface. (a,b) Shapes of water (a) and ammonia (b) molecules according to the VSEPR theory. Yellow clouds represent lone pairs of electrons in these molecules; arrows show the directions of the net dipole moments. (c) Idealized pictures of how the orientation of the molecular dipoles at the graphene/BTO interface translates into the polarization of BTO. (d,e) Orientations of the water molecules at the graphene/BTO interface for the cases when BTO is polarized downwards (d) and upwards (e). (f,g) Orientations of the ammonia molecules at the graphene/BTO interface for the cases when BTO is polarized downwards (d) and upwards (e). Figure 3: Differences in the alignment of water and ammonia molecules at the graphene/BTO interface. ( a , b ) Shapes of water ( a ) and ammonia ( b ) molecules according to the VSEPR theory. Yellow clouds represent lone pairs of electrons in these molecules; arrows show the directions of the net dipole moments. ( c ) Idealized pictures of how the orientation of the molecular dipoles at the graphene/BTO interface translates into the polarization of BTO. ( d , e ) Orientations of the water molecules at the graphene/BTO interface for the cases when BTO is polarized downwards ( d ) and upwards ( e ). ( f , g ) Orientations of the ammonia molecules at the graphene/BTO interface for the cases when BTO is polarized downwards ( d ) and upwards ( e ). Full size image When BTO is polarized downwards, the positively charged H atoms of a water molecule coordinate with any two adjacent oxygen atoms on the negatively charged BTO surface ( Fig. 3d ). As a result, the net dipole moment of water points to the same direction (downwards) as the polarization of BTO, as shown in Fig. 3c (top panel). This leads to a stable ferroelectric polarization due the negative polarization charge being stabilized by positively charged hydrogen atoms of H 2 O molecules. The situation changes markedly when the BTO is polarized upwards giving rise to the positive surface polarization charge. Since the ionic radius of Ti 4+ is much smaller than that of O 2− , the distance between the closest Ti atoms (~4 Å) on the barium titanate surface is much larger than the H–H distance in the water molecule (~1.5 Å). Hence, only one of two lone pairs of the water molecules coordinates with a Ti atom and water dipoles assume the orientation schematically shown in Fig. 3e . (This schematic also takes into consideration the fact that the oxygen atoms on the BTO surface attract hydrogen atoms and repel the farthest lone pair.) As a result, the dipole moment of the water molecule has a much stronger in-plane component leading to a polarization discontinuity at the H 2 O/BTO. In other words, switching of the BTO polarization from the downward to the upward direction does not translate into the reversal of the water dipoles, which explains why the upward polarization in the Gr/H 2 O/BTO junctions is unstable. On the other hand, in the Gr/NH 3 /BTO junctions, polarization reversal of the BTO layer always leads to flipping of the ammonia molecules so that their net dipole moments always point in the same direction as the polarization of BTO, as indicated in Fig. 3c . If the BTO layer is polarized downwards, the H atoms in the ammonia coordinate with negatively charged oxygen ions on the BTO surface, and the net dipole moment of the molecule also points downwards ( Fig. 3f ). If the BTO layer is polarized upwards, the only lone pair of the ammonia coordinates with positively charged Ti ions, and the net dipole moment of the molecule also points upwards ( Fig. 3g ). This realignment of the ammonia molecules provides strong retention for both upward and downward polarization states in the Gr/NH 3 /BTO junctions. Note, that since both ammonia and water are polar molecules of comparable size and relatively large dipole moments (1.47 D and 1.85 D, respectively), it could have been expected that they would have a similar effect on polarization stability. It appears that the size and polarity arguments alone are not sufficient, and more subtle geometrical differences between the molecules could result in substantial differences in their experimentally observed behaviour. While the organic molecules are unlikely to be compatible with the solid-state memory technology, the obtained results show that an active polar interfacial layer is a critical component, which can be used to enhance the functional behaviour (retention and resistive switching) of the FTJs. These devices could employ, for example, polarizable oxides at the interfaces, making this interface engineering approach much more amenable to the solid-state technology. In addition to the enhancement of the polarization stability, the ML between graphene and BTO plays an important role in the enhancement of the observed TER effect. As was discussed in ref. 32 , in the FTJ with a composite ferroelectric/dielectric barrier, due to a change in the electrostatic potential with polarization reversal caused by not fully screened depolarizing field, the dielectric layer acts as a switch that changes its barrier height from a low to a high value. We model this effect using a free-electron approach applied to a composite NH 3 /BTO barrier in the spirit of ref. 32 . The overall tunnelling potential profile seen by transport electrons is a superposition of the stepwise potential originating from the conduction band minimum and variation in the electrostatic potential resulting from the spontaneous polarization of the ferroelectric layer, the induced polarization in the ammonia dielectric layer and the screening charges in the electrodes. Our calculations show that for both polarization states the conductance per unit area, G/A, decreases exponentially with the NH 3 layer thickness t A ( Fig. 4a ). However, the slope of the calculated G/A( t A ) dependence is different for the two opposite polarizations of BTO, reflecting different heights of the electronic potential barrier (insets in Fig. 4a ) and consequently a different decay constant. As a result, the TER ratio increases exponentially with the ammonia layer thickness ( Fig. 4b ). For the NH 3 layer thickness of about 1 nm found from our experiment ( Supplementary Figs 7 and 8 ; Supplementary Note 5 ) and parameters used in the model (see Methods), the predicted values of the resistance-area product and OFF/ON ratio are in agreement with the experiment values. We note that similar to our previous work [5] , we find that ‘holes’ dominate the tunnelling mechanism. This behaviour is expected if the decay constant of the evanescent state in the tunnelling barrier is increasing with energy, which is the case for the Δ 1 band in BTO [33] . 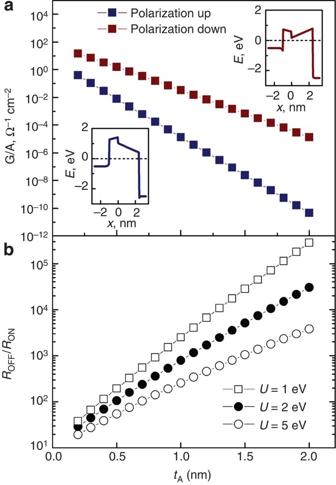Figure 4: Theoretical modelling of the electroresistance effect in the FTJ with a composite Gr/BTO barrier. (a) Calculated conductance per area (G/A) as a function of ammonia barrier thickness (tA) for polarization pointing up (blue) and down (red) and ammonia barrier heightUA=1 eV. Insets show the effective potential profile across the tunnel junction for polarization up (bottom inset) and down (top inset). Here the region of −1 nm<x<0 represents the ammonia interlayer and the region of 0<x<2.4 nm corresponds to the BaTiO3ferroelectric layer. (b)ROFF/RONresistance ratio as a function oftAforUA=1 eV (open squares),UA=2 eV (solid circles) andUA=5 eV (open circles). Figure 4: Theoretical modelling of the electroresistance effect in the FTJ with a composite Gr/BTO barrier. ( a ) Calculated conductance per area ( G / A ) as a function of ammonia barrier thickness ( t A ) for polarization pointing up (blue) and down (red) and ammonia barrier height U A =1 eV. Insets show the effective potential profile across the tunnel junction for polarization up (bottom inset) and down (top inset). Here the region of −1 nm< x <0 represents the ammonia interlayer and the region of 0< x <2.4 nm corresponds to the BaTiO 3 ferroelectric layer. ( b ) R OFF / R ON resistance ratio as a function of t A for U A =1 eV (open squares), U A =2 eV (solid circles) and U A =5 eV (open circles). Full size image Using graphene as an electrode in FTJs not only results in the enhanced performance of FTJs themselves but also reveals a new potential for graphene as a functional material. Most of the experiments so far were focused on using graphene in field-effect transistors, where the in-plane transport is modulated by a gate voltage. However, a sufficient OFF/ON current ratio in the graphene-based transistors with conventional device structures was not possible to obtain. Recently, a very large modulation on the device current (OFF/ON ratio of 10 5 ) has been achieved by adjusting the gate voltage to control the graphene–silicon Schottky barrier [34] . Our work demonstrates another example where graphene is used in a device with perpendicular-to-the-plane transport. The novelty of our approach is in exploiting the non-volatile nature of ferroelectric polarization states, which may have important implications in non-volatile memories and logic. Although modulation of the electronic properties of graphene did not contribute to the TER effect in the current experiments, additional modulation of graphene doping by electrical gating might further boost the electroresistance behaviour. This may be an interesting subject for future research. Sample preparation Epitaxial single-crystalline BTO films with thickness of 6 u.c. have been grown by pulsed laser deposition on atomically smooth TiO 2 -terminated (001)-STO substrates with a 30-nm-thick LSMO layer as a bottom electrode. Before deposition, low-angle miscut (<0.1°) STO substrates were etched using buffered hydrofluoric (HF) acid for 60 s to maintain Ti-termination and then were annealed in oxygen at 1,000 °C for 6 h to create atomically smooth surfaces with single-unit-cell-height steps. During deposition of all the layers substrate temperature was maintained at 680 °C with chamber oxygen pressure kept at 150 mTorr. The samples were cooled down to room temperature in oxygen atmosphere at 1 atm. Graphene films have been grown by the CVD in a home-built CVD system on 25-μm-thick Cu foils (Alfa Aesar). The foils were initially cleaned in acetic acid for 10 min, dried and annealed in H 2 at 1,000 °C for 30 min. Graphene growth has been performed at 1,000 °C for 20 min in a CH 4 :H 2 (1:1) atmosphere at 550 mTorr. The resulting graphene films were monolayer, which was confirmed by Raman spectroscopy ( Supplementary Fig. 1 ). To fabricate graphene patches, a graphene film was first transferred onto a silicon wafer with a 300-nm-thick SiO 2 surface layer (Silicon Quest International). To do this, 4% solution of 950 K PMMA solution in anisole was spin-coated on one side of a rectangular-shaped piece (~8 × 10 mm 2 ) of a graphene-covered Cu foil and dried for 20 min at room temperature. Then the foil was placed on the surface of 1 M HNO 3 and kept there for 5 min to remove graphene from the unprotected side and later transferred to a hot (60 °C) 1-M FeCl 3 aqueous solution to etch away the copper. The free transparent film was transferred on Si/SiO 2 wafer, dried and washed in a hot (50–60 °C) acetone bath, leaving single-layer graphene attached to the wafer. To fabricate graphene patches, the PMMA solution in anisole was spin-coated on Gr/SiO 2 /Si wafer and 10 × 30-μm 2 strips were patterned by electron beam lithography. The unprotected graphene was etched away by O 2 reactive ion etching (Trion Minilock Phantom III system). Then the wafer was placed on the surface of 5% HF solution (Alfa Aesar) and kept there for 3 min to etch away the SiO 2 layer. Transparent graphene/PMMA patches were then washed in distilled water and transferred on the surface of a BTO wafer. For NH 3 samples, graphene/PMMA patches were kept on the surface of NH 3 solution for 10 min before transferring on BTO. After drying at room temperature, the sample was exposed to acetone vapour to soften the polymer. After that the sample was washed twice in a hot (50–60 °C) acetone bath to remove PMMA. The reference Gr/BTO/LSMO junctions have been prepared by mechanical exfoliation of highly oriented pyrolytic graphite using adhesive Scotch tape [19] followed by transfer onto the surface of annealed BTO/LSMO substrates. This method does not use any media for transfer, which minimizes the chemistry effect at the interface between graphene and BTO. Characterization Polarization imaging and local switching spectroscopy has been performed using a resonant-enhanced PFM (MFP-3D, Asylum Research). Conductive silicon cantilevers (PPP-EFM, Nanosensors) have been used in this study. PFM hysteresis loops were obtained at fixed locations on the junction surface as a function of switching pulses (12 ms) superimposed on a.c. modulation bias with an amplitude of 0.6 V p-p at about 320 kHz. Tip contact forces have been calibrated by measuring force–distance curves and have been kept at a level of 20 nN. The Raman spectra were collected using a Thermo Scientific DXR Raman microscope with a 532-nm excitation laser. The X-ray photoelectron spectroscopy (XPS) was performed using an PHI Quantera SXM scanning X-ray microprobe. XPS measurements confirmed the presence of ammonia molecules at the interface between graphene and BTO (see Supplementary Figs 9 and 10 ). Details of the spectroscopic characterization of the interfacial ML in the Gr/NH 3 /BTO junctions can be found in Supplementary Note 6 . Modelling We describe LSMO and graphene electrodes within a free-electron model by the band filling, which is determined by a position of the Fermi energy E F with respect to the bottom of the conduction band E C . As representative values we assume E F − E C =2.5 eV for LSMO and E F − E C =0.5 eV for graphene. Electronic properties of ammonia are characterized by the energy gap between the LUMO and HOMO states of about 10 eV [35] . For the Fermi energy lying in the middle of the gap, the effective potential barrier produced by ammonia is U A =5 eV. We also performed a calculation for lower barrier heights of U A =2 eV and U A =1 eV. For the dielectric constant of ammonia we use ε A =17 as a representative value at room temperature [36] . The parameters of BTO are assumed to be similar to those used previously [37] , namely, the ferroelectric barrier height U f =0. 6 eV, dielectric constant ε f =80 and polarization P =20 μC cm −2 . To calculate the electrostatic potential, we employ the Thomas–Fermi model of screening and impose short-circuit boundary conditions. The computed screening lengths for top and bottom electrodes are about 0.2 nm for LSMO and 0.3 nm for graphene. The tunnelling conductance per unit area is calculated using the Landauer formula. The transmission coefficient is obtained from the solution of the Schrödinger equation by imposing a boundary condition of the incoming plane wave normalized to a unit flux density [32] . For the assumed parameters and the NH 3 layer thickness of 1 nm, the calculated values of the resistance-area product and TER are consistent with experiment values when U A =1 eV. How to cite this article : Lu, H. et al. Ferroelectric tunnel junctions with graphene electrodes. Nat. Commun. 5:5518 doi: 10.1038/ncomms6518 (2014).